Prediction and quantification of bioactive microbiota metabolites in the mouse gut Metabolites produced by the intestinal microbiota are potentially important physiological modulators. Here we present a metabolomics strategy that models microbiota metabolism as a reaction network and utilizes pathway analysis to facilitate identification and characterization of microbiota metabolites. Of the 2,409 reactions in the model, ~53% do not occur in the host, and thus represent functions dependent on the microbiota. The largest group of such reactions involves amino-acid metabolism. Focusing on aromatic amino acids, we predict metabolic products that can be derived from these sources, while discriminating between microbiota- and host-dependent derivatives. We confirm the presence of 26 out of 49 predicted metabolites, and quantify their levels in the caecum of control and germ-free mice using two independent mass spectrometry methods. We further investigate the bioactivity of the confirmed metabolites, and identify two microbiota-generated metabolites (5-hydroxy-L-tryptophan and salicylate) as activators of the aryl hydrocarbon receptor. The human gastrointestinal (GI) tract is colonized by ~10 14 microorganisms that are collectively termed the microbiota. Disruptions in the microbiota composition (dysbiosis) are increasingly correlated to not only gut diseases [1] , but also obesity, insulin resistance and type 2 diabetes [2] , [3] . There is increasing evidence that the functional outputs of the microbiota, that is, the metabolites they produce, are important modulators of host physiology in the GI tract. Work from our laboratory [4] and another group [5] demonstrated that the tryptophan (Trp)-derived bacterial metabolite indole attenuates indicators of inflammation and improves tight junction properties in intestinal epithelial cells in vitro and in vivo . Fukuda et al. [6] reported that acetate produced by intestinal bacteria inhibits translocation of E. coli O157:H7 Shiga toxin from the gut lumen to systemic circulation. Other short-chain fatty acids such as butyrate and propionate have been shown to induce the differentiation of naive T cells into anti-inflammatory regulatory T cells (T reg ) [7] , and into Th1 and Th17 T cells that also produce interleukin (IL)-10 (ref. 8 ). Despite a high level of interest, only a handful of bioactive microbiota metabolites in the GI tract have been identified. One major challenge is that the spectrum of metabolites present in the GI tract is extremely complex, as the microbiota can carry out a diverse range of biotransformation reactions, including those that are not present in the mammalian host [9] . Isolating and culturing individual bacterial species to identify the metabolites produced in these cultures remain challenging, as many intestinal bacteria cannot be cultured under standard laboratory conditions. Moreover, this approach does not account for community-level interactions between the microorganisms as metabolites produced by one microorganism can be utilized or modified by other microorganisms. Another challenge lies in classifying a metabolite as either microbiota- or host-derived, as many metabolites are present in both microorganisms and mammals because of the high degree of conservation of metabolic pathways across organisms [10] . Metabolomics of faecal or body fluid samples has been increasingly used to explore the metabolite profiles of the GI tract, and to compare these profiles under different physiological or disease conditions. Mass spectrometry (MS)-based untargeted approaches have been especially useful in analysing a broad spectrum of metabolites in a high throughput manner [11] . While this approach offers the benefit of potential for discovery, it also has drawbacks. Owing to the complexity of the mass spectra obtained from full-scan experiments, metabolite identification can be difficult, especially if neither high purity standards nor database entries are available for the metabolites of interest. High-resolution time-of-flight (TOF) mass spectrometers can somewhat alleviate this problem [12] , as chemical identities can be established based on exact mass as well as isotope and MS/MS fragmentation patterns. Alternatively, targeted analysis of an a priori selected set of metabolites affords custom optimization of MS parameters for individual metabolites to enable sensitive detection using quantitative methods such as multiple reaction monitoring (MRM). The obvious drawback is that the discovery potential can be limited. Importantly, neither untargeted nor targeted metabolomics can determine whether a gut metabolite is the product of host or microbiota metabolism as a standalone approach, as many metabolites can be produced in both mammalian and bacterial cells. In this work, we present a targeted approach that addresses the discovery limitation by integrating an in silico prediction step into the metabolomics workflow. To date, bioinformatics tools have been utilized in metabolomics generally for post hoc analysis to process data [13] or perform statistical comparisons [14] . Recently, Greenblum et al. [15] presented an elegant metagenomic study that places obesity- or inflammatory bowel disease (IBD)-associated variations in human gut microbiota gene abundances in the context of a microbial community-level metabolic network. The present study similarly models microbiota metabolism as a reaction network and uses this model to computationally explore the products of microbiota metabolism from aromatic amino acids (AAAs). We thus exploit efficient algorithms for network analysis and the growing catalogue of annotated microbial genomes to conduct in silico discovery experiments. Specifically, we utilize a probabilistic pathway construction algorithm to identify potential derivatives of AAAs while discriminating between microbiota and host contributions to the formation of the derivatives. To validate our methodology, we predict and experimentally analyse both bacteria- and host-derived products of aromatic amino acids (AAAs). We utilize two independent MS methods to quantify the levels of the predicted metabolites in caecum contents from conventionally raised specific pathogen-free (SPF) and germ-free (GF) mice. On the basis of recent studies suggesting that AAA-derived metabolites could be potent aryl hydrocarbon receptor (AhR) ligands in the context of host immune system function [16] , mucosal reactivity [17] and oxidative stress defense [18] , we use a Gaussia luciferase (GLuc) reporter system to monitor the ability of the identified metabolites to activate the AhR. The workflow described in this study maps the identified metabolites to specific metabolic pathways, which can then be traced to the corresponding genes and species harbouring the genes, thereby facilitating the elucidation of functional contributions by the microbiota to the complex metabolite profile of the gut. Diversity and uniqueness of microbiota metabolic functions A combined host–microbiota reaction network model of gut microbiota metabolism was constructed based on genome annotation information on select bacteria reported to be present in the human GI tract [19] . The model comprises 3,449 distinct reactions, of which 940 are unique to the host, 1,267 are unique to the gut microbiota and 1,142 are present in both ( Fig. 1 ) [20] . Certain metabolic functions, for example, lipopolysaccharide biosynthesis, are dominated by reactions only present in the microbiota ( Fig. 1 , i). In contrast, other functions, such as steroid biosynthesis, are performed by the host without the involvement of bacterial species in the microbiota ( Fig. 1 , ii). Overall, this type of exclusivity is the exception, rather than the rule, as the majority of functions (61 out of 82 categories) include both host- and microbiota-specific reactions. 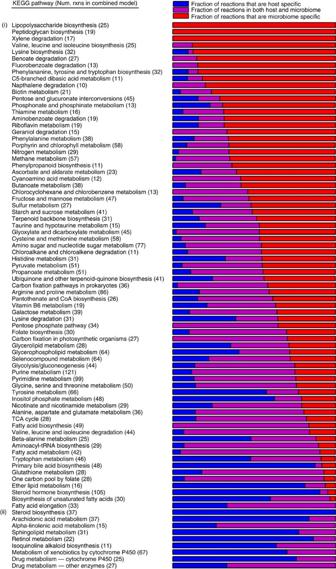Figure 1: Function categories of reactions in the combined microbiota–host model. Colours indicate whether the reactions are host-specific, microbiome-specific or are present in both. The length of each coloured segment is proportional to the fraction contributed by the corresponding system (host, microbiota or both). Figure 1: Function categories of reactions in the combined microbiota–host model. Colours indicate whether the reactions are host-specific, microbiome-specific or are present in both. The length of each coloured segment is proportional to the fraction contributed by the corresponding system (host, microbiota or both). Full size image To investigate the distribution of metabolic functions across different subsets of the microbiota, a phylum score was computed for each reaction characterizing its prevalence in different phyla. Out of the 2,409 reactions in the microbiota model, only 286 reactions belong to a single phylum ( Fig. 2a ). The most conserved function is translation, with 83% of the reactions present in all five bacterial phyla comprising the microbiota model. Interestingly, the least conserved function category is energy metabolism, with only 13% of the reactions present in all five phyla. The number of reactions in each function category also varied substantially depending on the function. The largest number of reactions (493 out of 2,409) belongs to a category designated as ‘unclassified’ by KEGG. The largest category with an assigned function is amino-acid metabolism, accounting for 16% of all reactions in the microbiota model. Proteobacteria possess the broadest coverage of amino-acid reactions, expressing genes for 349 of the 392 amino-acid reactions in the microbiota model. Approximately 9% of the amino-acid reactions are unique to this phylum, which is greater than the number of amino-acid reactions unique to the other four phyla combined. 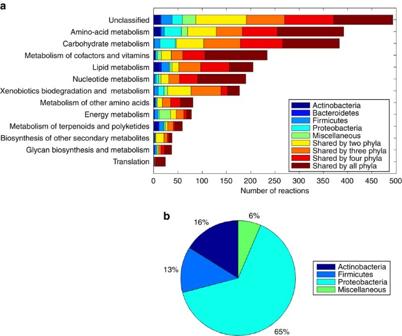Figure 2: Distribution of functional categories across microbiota. (a) Function categories of reactions in the gut microbiota model and their uniqueness determined at the phylum level. Uniqueness was determined based on the phyla score (see Methods). (b) Distribution of unique reactions involved in aromatic amino-acid metabolism. Figure 2: Distribution of functional categories across microbiota. ( a ) Function categories of reactions in the gut microbiota model and their uniqueness determined at the phylum level. Uniqueness was determined based on the phyla score (see Methods). ( b ) Distribution of unique reactions involved in aromatic amino-acid metabolism. Full size image Biotransformation of aromatic amino acids We focused on aromatic amino acids (AAAs), as several previous studies, including our own work [4] , suggested that these are putative precursors of bioactive bacterial metabolites. Out of the 169 AAA reactions in the combined host–microbiota model, the gut microbiota harbours 99 reactions, with 66 reactions not encoded by the host genome. A majority of these reactions are contributed by Proteobacteria ( Fig. 2b ), particularly Enterobacter and Escherichia . The KEGG function categories, while useful for broad assessment of metabolic capabilities, can be ambiguous. For example, tryptophan transaminase (EC no. 2.6.1.27) is assigned to tryptophan (Trp) metabolism, whereas indole-2-monooxygenase (EC no. 1.14.13.137) is assigned to benzoxazinoid biosynthesis, even though both enzymes are two steps from Trp. Visual inspection of the current KEGG map for Trp metabolism suggests that indole can only be converted to either indoxyl or 2-formylamino-benzaldehyde. However, indole can also be converted to indole-2-dione through the aforementioned monooxygenase. This example illustrates the need for a more systematic analysis. To this end, we searched for metabolites that are biochemically related to AAAs by constructing possible biotransformation pathways for Phe, Trp or Tyr, while discriminating between microbiota and host reactions. Pathway construction proceeded by selectively adding reactions only present in the microbiota, and terminated when no such reaction could be added. This ensured that none of the intermediates, except the terminal metabolite in the pathway, could be formed through a host reaction. Owing to the probabilistic nature of the pathway construction algorithm, the results could vary with the number of iterations. Therefore, we performed a series of simulations where we varied the iteration numbers until we did not observe any further increase in the number of unique pathways ( Supplementary Fig. 1 ). For Trp, this probabilistic search returned three pathways composed of strictly bacterial enzymes ( Fig. 3 ). The remaining single-step ‘pathways’ represent the termination steps enforced by the algorithm’s stopping criterion. The total number of Trp derivatives identified in this way is 10. Of these, the following four compounds only participate in microbiota metabolism, per KEGG’s annotation: indole, indoleglycerol phosphate, 1-(2-carboxyphenylamino)-1-deoxy-D-ribulose 5-phosphate and N-(5-phospho-D-ribosyl) anthranilate. The remaining metabolites participate in both microbiota and host metabolism. For phenylalanine (Phe), the search returned 12 distinct pathways composed of strictly bacterial enzymes, and three pathways composed of enzymes expressed in both the microbiota and host ( Supplementary Fig. 2 ). Of a total of 33 predicted derivatives, 21 participate only in microbiota metabolism, whereas 11 participate in microbiota and host reactions ( Supplementary Table 1 ). Finally, the search on tyrosine (Tyr) returned only one bacterial pathway ( Supplementary Fig. 3 ), as all other reactions directly connected to Tyr were present in the host. 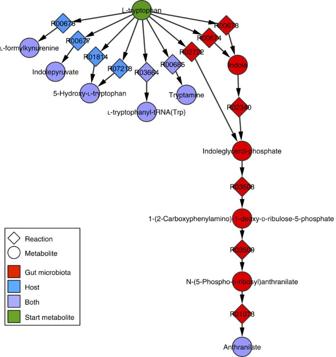Figure 3: Metabolic derivatives of tryptophan (Trp) identified from probabilistic pathway construction. Starting with Trp, pathways were constructed by recursively adding a reaction and then checking whether the reaction is present in the host. The tree diagram shown represents the union of all pathways identified in this way. As constrained by the algorithm, each branch of the tree terminates at a metabolite that is present in the host (blue or purple). Reaction numbers (for example, R00674) refer to KEGG IDs. Figure 3: Metabolic derivatives of tryptophan (Trp) identified from probabilistic pathway construction. Starting with Trp, pathways were constructed by recursively adding a reaction and then checking whether the reaction is present in the host. The tree diagram shown represents the union of all pathways identified in this way. As constrained by the algorithm, each branch of the tree terminates at a metabolite that is present in the host (blue or purple). Reaction numbers (for example, R00674) refer to KEGG IDs. Full size image Metabolite analysis We used a targeted metabolomics approach to measure the predicted panel of metabolites, including derivatives that form through reactions present in the host. Of the 49 predicted derivatives, a subset of 19 metabolites was analysed using MRM, taking into account availability of pure standards and ease of ionization and fragmentation. To broaden the scope of metabolic profiling, the predicted metabolites were also analysed using a second MS method, information-dependent acquisition (IDA). This method allowed detection and identification of additional metabolites based on accurate mass even when high-purity standards were unavailable. On the other hand, we found that the MRM method offered greater dynamic response and detection sensitivity for some metabolites ( Supplementary Fig. 4 ). The final panel of metabolites targeted for MRM and IDA analyses is listed in Supplementary Table 1 . For MRM analysis, metabolite identification was performed based on both chromatographic retention time and mass signature, as we found that even an optimized MRM transition (precursor–product ion pair) did not always uniquely identify a metabolite in a complex biological sample ( Supplementary Fig. 5 ). For IDA analysis, the identity of a detected metabolite was determined based on accurate mass and isotope pattern, and, whenever possible, confirmed based on measured MS/MS fragmentation patterns. As pure chemical standards were not used for the IDA experiments, the metabolite concentrations are reported in terms of total ion counts normalized to mass of caecal contents. Combined, the two methods detected 26 of the 49 predicted metabolites in the caecal contents of (conventionally raised) SPF or GF mice ( Supplementary Table 1 ). Of the detected metabolites, 16 metabolites only participate in microbiota-specific reactions according to KEGG’s annotation, whereas the remaining 10 participate in reactions present in both the microbiota and host ( Fig. 4 ). We did not detect any metabolites that only participate in host-specific reactions. In the subset of 23 metabolites that was not detected, the number of microbiota- and host-specific metabolites was eight and four, respectively, with the remaining eleven participating in reactions present in both the microbiota and host. Taken together, these trends suggest that a host-specific AAA derivative is less likely to be present in the caecal contents than a derivative that could form through reactions present in the microbiota. Furthermore, we found that more than half (15/26) of the detected metabolites were either significantly reduced or absent in GF mice ( Fig. 5 ), corroborating the contribution of intestinal microbes to the presence of these metabolites. 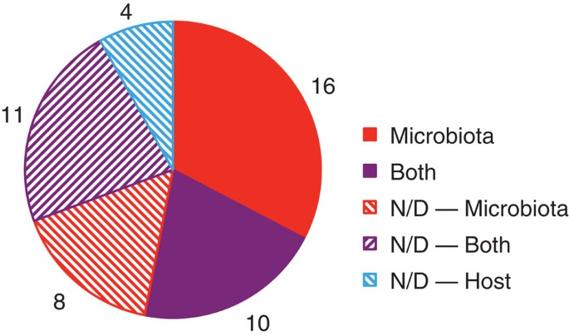Figure 4: Summary of predicted and detected metabolites. A metabolite was classified as microbiota, host or both based on whether a reaction involving the metabolite is microbiota-specific, host-specific or expressed in both the microbiota and host per KEGG annotation. Solid and shaded pies represent metabolites that were detected and not detected (N/D), respectively. Figure 4: Summary of predicted and detected metabolites. A metabolite was classified as microbiota, host or both based on whether a reaction involving the metabolite is microbiota-specific, host-specific or expressed in both the microbiota and host per KEGG annotation. Solid and shaded pies represent metabolites that were detected and not detected (N/D), respectively. 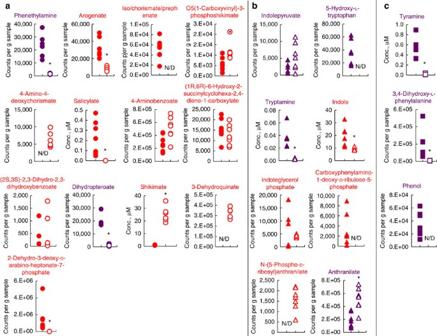Figure 5: Comparison of metabolite concentrations in caecum luminal contents from SP and GF mice determined using MRM and IDA MS. Metabolite concentrations (MRM) and counts (IDA) were normalized to the corresponding wet weight of caecal contents. Circles (a), triangles (b) and squares (c) denote Phe, Trp and Tyr derivatives, respectively. Colours indicate whether the metabolite participates only in microbiota metabolism (red) or both host and microbiota metabolism (purple). Host-specific metabolites were not detected. Closed and open symbols denote samples from SPF and GF mice, respectively. Isochorismate, chorismate and prephenate are all represented in the same plot as they have identical exact masses. An asterisk (*) indicates a statistically significant difference between the GF and SPF groups (two-sided Mann–WhitneyU-test,P<0.05). N/D: not detected. Full size image Figure 5: Comparison of metabolite concentrations in caecum luminal contents from SP and GF mice determined using MRM and IDA MS. Metabolite concentrations (MRM) and counts (IDA) were normalized to the corresponding wet weight of caecal contents. Circles ( a ), triangles ( b ) and squares ( c ) denote Phe, Trp and Tyr derivatives, respectively. Colours indicate whether the metabolite participates only in microbiota metabolism (red) or both host and microbiota metabolism (purple). Host-specific metabolites were not detected. Closed and open symbols denote samples from SPF and GF mice, respectively. Isochorismate, chorismate and prephenate are all represented in the same plot as they have identical exact masses. An asterisk (*) indicates a statistically significant difference between the GF and SPF groups (two-sided Mann–Whitney U -test, P <0.05). N/D: not detected. Full size image Only a small fraction (3/25) of the detected metabolites—shikimate, tryptamine and tyramine—could be analysed by both MRM and IDA, with the latter method providing broader coverage (24 versus 6 metabolites detected by IDA and MRM, respectively). For the three metabolites detected by both methods, the results were consistent. Shikimate was dramatically reduced, whereas tryptamine and tyramine were significantly increased in SPF samples compared with GF samples ( Supplementary Fig. 6 ). For metabolites detected in both SPF and GF samples and significantly reduced in the GF condition, the fold-changes ranged from ca. 2 to 300. For Trp, two of the four intermediates comprising the longest microbiota pathway ( Fig. 3 ) were reduced or altogether absent in GF samples. Indole was reduced 2.2-fold, whereas 1-(2-Carboxyphenylamino)-1-deoxy- D -ribulose-5-phosphate was not detected in GF samples. For Phe, major branch points of the microbiota pathways occur at chorismate and isochorismate. The intermediates upstream of these branch points are, in order, arogenate and prephenate ( Supplementary Fig. 2 ). All four microbiota metabolites were reduced ( ca. 3.6-fold in the case of arogenate) or not detected in GF samples. Downstream of these two branch points, the trends were mixed, as some intermediates, notably those of the shikimate branch, were only detected in GF samples. For Tyr, all three detected metabolites were significantly reduced in GF samples ( Fig. 5 ). Activation of AhR by microbiota metabolites In order to link the in vivo presence of the AAA-derived metabolites to the regulation of host function, we investigated whether the metabolites detected in the caecal contents could activate an eukaryotic signalling pathway. As we were interested in establishing the bioactivity of specific metabolites, we confined the analysis to nine metabolites (5-hydroxy-L-tryptophan, indole, indolepyruvate, salicylate, shikimate, tryptamine, chorismate, 3,4-dihydroxyl- L -phenylalanine and tyramine) that could be obtained as high-purity chemicals from a commercial source. We focused on the AhR as recent studies have highlighted the importance of this receptor in regulating gut physiology [21] , [22] , [23] . Furthermore, previous studies [24] have shown that endogenous Trp-derived metabolites such as kynurenine (host-derived) and 6-formylindolo[3,2-b]carbazole (an ultraviolet-exposed Trp degradation product) are potent ligands for AhR [25] . Therefore, we investigated whether microbiota metabolites derived from AAAs are ligands for the AhR. We used MCF-7 (Michigan Cancer Foundation-7) human breast cancer cells as the model cell line, as prior work has shown high levels of AhR responsiveness in these cells [26] . MCF-7 cells with a stably integrated GLuc reporter plasmid for AhR-binding activity were exposed to microbiota metabolites or 20 nM 2,3,7,8-tetrachlorodibenzo- p -dioxin (TCDD; xenobiotic-positive control that is an AhR ligand) for 48 h, and luciferase activity in culture supernatants was measured. Kynurenine, an endogenous AhR ligand derived from Trp by host indoleamine 2,3-dioxygenase activity [27] , was used as an additional positive control. Exposure to 20 nM TCDD and 100 μM kynurenine resulted in a 3.9- and 2-fold increase in the rate of AhR-driven luciferase activity (relative light unit (RLU)/h/relative fluorescence unit), respectively, as compared with the solvent control ( Fig. 6 ). Of the nine metabolites tested, five metabolites (5-hydroxy-L-tryptophan, indolepyruvate, tryptamine, salicylate and shikimate) induced AhR activity in MCF-7 cells ( Fig. 6 ). Depending on the metabolite, the lowest concentration that could stimulate significant AhR activity varied over several orders of magnitude. For example, 5-hydroxy-L-tryptophan induced AhR activity at 0.01 μM, whereas indolepyruvate required a concentration greater than 100 μM to show significant activity. The minimum concentration needed to activate the AhR for the other metabolites fell within this range, with salicylate and shikimate inducing activity at 10 μM and tryptamine at 100 μM. 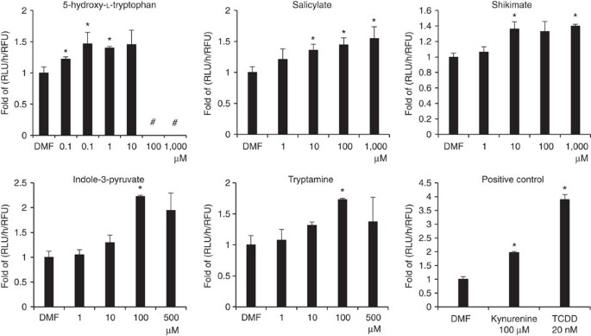Figure 6: Dose-dependent activation of the AhR by AAA-derived metabolites. AhR activity is reported as the rate of luciferase activity normalized to red fluorescence of constitutively expressed RFP (RLU/h/relative fluorescence unit (RFU)). Positive controls were 20 nM TCDD and 100 μM kynurenine, and the negative control was 0.1% (v/v)N, N-dimethylformamide. Data shown are mean±s.d. from four replicate experiments. Asterisk (*) indicates statistical significance atP<0.05 using the Student’st-test. Results for 100 μM and 1000 μM 5-hydroxy-L-tryptophan are marked with # as cell death was observed at these concentrations. Figure 6: Dose-dependent activation of the AhR by AAA-derived metabolites. AhR activity is reported as the rate of luciferase activity normalized to red fluorescence of constitutively expressed RFP (RLU/h/relative fluorescence unit (RFU)). Positive controls were 20 nM TCDD and 100 μM kynurenine, and the negative control was 0.1% (v/v) N, N -dimethylformamide. Data shown are mean±s.d. from four replicate experiments. Asterisk (*) indicates statistical significance at P <0.05 using the Student’s t -test. Results for 100 μM and 1000 μM 5-hydroxy- L -tryptophan are marked with # as cell death was observed at these concentrations. Full size image We present here a methodology for the identification of gut microbiota metabolites that integrates computational pathway analysis into a targeted metabolomics workflow. We predicted and profiled possible biotransformation products of AAAs (Trp, Phe and Tyr), and detected a majority (26 out of 49) of the predicted metabolites in caecal contents from mice. All of the detected metabolites could be formed through bacterial reactions from one of the source amino acids, none of these metabolites were host-specific, and a majority (15 out of 26) of the detected metabolites were significantly reduced in GF mice relative to SPF mice. The effects of physiological or pathological perturbations on the intestinal microbiota have been investigated using metagenomic analyses characterizing the composition of the gut microbial community, the enrichment (or depletion) of bacterial genes or the expression levels of genes for specific metabolic pathways [28] , [29] , [30] . A limitation of these analyses is that they do not provide direct information on which molecules are formed from which bacterial biotransformation reactions and which metabolic products are increased or decreased under different conditions. Thus, the ability to unambiguously identify and quantify bacterial metabolites is expected to have a significant impact on the study of human gut microbiome function. One obvious qualification in interpreting the in silico analysis is that the reliability of our model is predicated on the accuracy of the annotation in the reaction database (in our case KEGG). While the KEGG database is continually updated, it is certainly possible that there are missing entries or incorrect annotations, which could explain why the predictions were not 100% accurate. For example, Wikoff et al. [31] identified indole-3-propionate as a Trp-derived metabolite that is produced by the gut microbiota. However, at the time of completion of this work, this metabolite was not listed in the KEGG Compound database, and thus could not be identified by our algorithm. Similarly, the discrimination of bacterial metabolites from metabolites that could also be produced by host cells depends on an accurate model of host metabolism. The most relevant host genomes, for example, mouse and human, have been sequenced and largely annotated, and several published genome-scale model reconstructions exist. However, prior studies suggest that several iterations may be required [32] until a published model can be considered a stable, consensus reconstruction [33] . Currently, there is no consensus model of gut microbiota metabolism. One approach has been to build species-specific genome-scale models, and apply constrained optimization methods such as flux balance analysis to characterize the metabolic capacities of the microbe. For example, Heinken et al. [34] utilized a genome-scale metabolic reconstruction of Bacteroides thetaiotaomicron in conjunction with flux balance analysis to explore the co-metabolism between a commensal microbe and its murine host, reporting that the microbe could rescue a potentially lethal loss of enzymatic function in the host. More recently, Shoaie et al. [35] assembled metabolic reconstructions of three species, Eubacterium rectale , Methanobrevibacter smithii and B. thetaiotaomicron , as representatives of three main phyla in the human gut, which were used to simulate the metabolic interactions between the species under varying nutrient settings. An alternative approach is to treat the microbiota as a single ‘super’ organism and model the metabolic capability of the microbiota at the community level. This approach has the drawback that interactions between particular species cannot be examined in detail. However, such community-level models can be directly applied to the growing volume of metagenomic data to comprehensively analyse the diversity of metabolic functions collectively encoded by the GI microbiome [36] , [37] . Recently, Greenblum et al. [15] assembled a community-level model of human GI tract microbiota to find significant alterations in the functional organization of the microbiota metabolic network in obesity and IBD. We also modelled the microbiota as a unified system, abstracting the union of all enzymes collectively encoded by the different species as part of a single reaction network. As one of our goals was to discriminate between microbiota and host products of metabolism, we extended this community-level analysis by also assembling a host metabolic model, and utilizing this model to identify the metabolic functions that depend on the microbiota. Although our study uses the mouse as the model host organism, the microbiota model was constructed from microbiome data on the human intestine because the list of documented intestinal bacteria is more extensive for humans than mice. However, a recent meta-analysis showed that mice and human gut microbiota share a very strong similarity (90% and 89% of bacterial phyla and genera, respectively) [38] , and that the most abundant bacterial species are common to human and murine gut microbiota. Therefore, we assumed that a sampling of the most common species found in the human GI tract should reasonably approximate the biochemical diversity of the murine gut microbiota. We evaluated the pathway analysis results from the combined microbiota–host model by performing targeted metabolomics experiments, focusing on AAAs. These amino acids can be endogenously transformed into a variety of bioactive derivatives formed by commensal bacteria in the intestine (for example, indole from Trp [4] ). In the present study, we used a probabilistic pathway construction algorithm to identify metabolic derivatives that can be produced from Trp, Phe or Tyr via enzymatic reactions, while also mapping the enzymes involved to the host or microbiota metabolic network. An alternative approach would be to exhaustively search through the combined microbiota–host network to build a subnetwork comprising all reactions and metabolites that connect to a source metabolite, similar to the ‘scope’ analysis described in ref. 39 . This approach would confer a speed advantage over pathway construction, if the goals were to simply enumerate all possible metabolites that are connected to the source metabolite via enzymatic reactions. However, this approach does not provide information on the composition of pathways that connect a particular biotransformation product to a specific source metabolite. This information is necessary to determine whether the formation of the biotransformation product requires any microbial enzymes. Moreover, the set of metabolites resulting from network expansion may not resemble the starting metabolite in a meaningful way. For example, Trp can be converted to glucose and ketone bodies, which in turn can be further oxidized through the main pathways of central carbon metabolism. Therefore, a pathway analysis-based approach that avoids these issues is desirable. The algorithm used in this study can efficiently sample pathways connected to a source metabolite of interest, while shaping pathway construction through the reaction selection criteria. Directing the algorithm to only select reactions that are absent in the host when constructing a biotransformation pathway ensured that the intermediates would not be connected to other metabolites in the host metabolic network, and thus can be unambiguously designated as products of microbiota metabolism. This search strategy also avoided the enumeration of common hub metabolites that are the intermediates of central carbon pathways such as TCA cycle and glycolysis, which are found in all living cells. A potential drawback, however, is that this type of pathway construction cannot fully reflect host–microbiota co-metabolism; that is, certain biotransformation products that require multiple reactions expressed in both microbiota and host cannot be identified in this way. One way to address this issue is to simply restart pathway construction at a terminal metabolite node. For example, restarting the search at indolepyruvate extends this branch by adding a bacterial reaction producing indole-3-acetaldehyde, before terminating with a reaction present in both host and microbiota that produces indole-3-acetate ( Supplementary Fig. 7a ). Since formation of indolepyruvate requires a host-specific enzyme, indole-3-acetaldehyde and indole-3-acetate can be considered products of host–microbiota co-metabolism. Using MRM analysis, we found that GF caecum samples contained 30-fold less indole-3-acetate compared with SPF samples ( Supplementary Fig. 7b ), consistent with our analysis that production of this metabolite depends on the microbiota, and highlighting the utility of our approach for determining host–microbiota co-metabolism. A second way to explore host–microbiota co-metabolism is to search exhaustively, where pathway construction can utilize all reactions in the combined host–microbiota model, and then post process the search results using annotation data to identify metabolic products that are downstream of at least one microbiota reaction. We explored this idea by limiting the pathway length to four reactions from the source metabolite to keep computational runtime to within hours. While we found 64,741 distinct paths for Trp, many of them do not describe a meaningful biotransformation of the source metabolite. For example, this analysis predicts chorismate as a Trp-derived metabolite; however, this pathway involves serine and pyruvate as intermediates, casting doubt that chorismate can be meaningfully classified as a Trp-derived product. It should be possible to circumvent this issue by pruning the results of the exhaustive search by filtering for a functional group that is characteristic of the source metabolite of interest. For example, imposing the constraint that every intermediary metabolite along a pathway must possess a six-carbon aromatic ring eliminates all but 87 paths. However, this type of filtering may not be generally applicable, since other classes of metabolites, for example, organic acids, may lack a distinctive characteristic functional group. Moreover, exhaustive pathway enumeration has an exponential runtime of k l , where k is the average number of reactions connected to a metabolite and l scales with the maximal pathway length. Increasing the length limit to more than four reactions would lead to runtimes that are on the order of days using a typical workstation. This demonstrates the value of a sampling-based approach for constructing pathways of arbitrary length, which involves a more manageable polynomial runtime with respect to the number of iterations. We found that both MRM and IDA have advantages and disadvantages for experimental evaluation of the computational analysis. An important benefit of MRM is that when high-purity standards are available, the selective detection of specific precursor–product ion pairs can enhance sensitivity and improve LOD. Instrument-specific parameters can be tailored and optimized for each individual MRM transition, whereas full-scan methods use a particular set of parameters for all analytes, which may be suboptimal for a subset of the metabolites. In practice, we found that even optimized MRM transitions may not represent a unique mass signature for a metabolite, as there are cases where multiple analytes present in a biological sample share the same transition with the highest intensity. For example, indole 3-acetamide shows a strong signal for the 175→130 transition, as does arginine, a highly abundant amino acid. Similarly, metabolites possessing thermally labile bonds can decompose at the ion source. For example, a pure sample of Trp showed a strong MRM signal for the indole transition (118→91) at the expected retention time for Trp ( Supplementary Fig. 5b ), which was presumably because of partial decomposition of Trp into indole by the heated electrospray ionization. In this study, we utilized high-resolution MS to identify metabolites based on accurate mass as an alternative to MRM MS when high-purity standards are not available. Specifically, we performed IDA experiments to collect full-scan MS data with very high mass accuracy, while monitoring the MS/MS spectra for all ions meeting a specified count threshold whenever fragmentation could be achieved. Differences in instrument design also contributed to a difference in sensitivity between the MRM and IDA experiments. A comparison of the signal versus concentration plot for Trp showed that IDA provides approximately one-tenth of the sensitivity of MRM ( Supplementary Fig. 4 ). In fact, certain metabolites such as indole and salicylate could not be detected at all in a biological sample using IDA, whereas they could be quantified using MRM. These examples suggest that the choice between MRM and IDA will have to balance a tradeoff between sensitivity and resolving power. To our knowledge, this is the first targeted metabolomics study to quantitatively estimate the physiological concentration of several microbiota-produced metabolites present in caecum contents. While the literature on absolute concentrations of microbiota metabolites is relatively sparse, we found good agreement between our results and previously reported values. In an early study, Whitt and Demoss [40] used an enzymatic assay to determine an indole concentration of ~40 nmol g −1 tissue in murine caecum, which is comparable to our results (10–40 nmol g −1 sample wet weight in SPF caecum). In addition, we detected and identified a number of metabolites using IDA for which pure standards were unavailable. While we could not obtain absolute concentrations for these metabolites, it was possible to determine fold-changes across GF and SPF samples ( Fig. 5 ). Our results on metabolite differences between SPF and GF mice are comparable to other previous studies. Zheng et al. [11] profiled urinary and faecal metabolites of Wistar rats exposed to β-lactam antibiotics and detected tryptamine, indole-3-acetate, indole, shikimate and phenol in urine, and tryptamine and tyramine in faeces, which we detected in the caecum in the present study ( Supplementary Table 1 ). They also observed that the levels of indole-3-acetate, indole and phenol were lower in the antibiotic-treated mice, presumably because of the effect of the antibiotic on the gut microbiota. These results are in agreement with the reduction in these metabolites we observed in GF caecal contents ( Fig. 5 ). Interestingly, Zheng et al. [11] reported that antibiotic exposure increased the level of shikimate relative to the control group, which is also consistent with our data. The trends in our data are also similar to those reported by Wikoff et al. [31] , who compared plasma metabolites from GF and conventionally raised (CONV) mice. This comparison found that indoxyl sulfate and indole-3-propionic acid were present in the plasma of CONV mice, but were absent in GF mice, which is consistent with our observations that indole is reduced in GF samples ( Fig. 5 ). Likewise, phenyl sulfate, a xenobiotic transformation product of phenol, was only detected in CONV mice, also in agreement with our results showing that phenol is absent in GF mice. Similarly, our observation that tyramine levels are reduced in GF caecal contents is consistent with the differences in the colonic luminal contents from GF mice relative to Ex-GF mice inoculated with a faecal suspension from SPF mice [41] . However, unlike our study, this comparison of GF and Ex-GF mice did not attempt to attribute changes in the metabolites to specific bacterial pathways. Instead, metabolites were grouped into host- or microbiota-contributed products solely based on their relative amounts in GF and Ex-GF samples. The AhR is a ligand-activated transcription factor that plays an important role in the mucosal immune system [42] . Earlier work has shown that the plant secondary metabolite indole-3-carbinol can bind and activate the AhR [43] . In our study, we observed that four of the Trp derivatives (5-hydroxy- L -tryptophan, indole-3-acetate, tryptamine and indolepyruvate) and two of the Phe derivatives (salicylate and shikimate) could activate the AhR in a dose-dependent manner ( Fig. 6 and Supplementary Fig. 7c ). To our knowledge, this is the first report identifying 5-hydroxy- L -tryptophan, salicylate and shikimate as non-host-derived activators for the AhR. Our results are also consistent with a previous study by Heath-Pagliuso et al. [24] , who showed that tryptamine and indole-3-acetate are AhR ligands. We found that five metabolites predicted to be microbiota-specific are significantly elevated in the GF samples, which is somewhat counterintuitive ( Fig. 5 ). Three of these metabolites, shikimate, 3-dehydroquinate and O5(1-carboxyvinyl)-3-phosphoshikimate, are intermediates of the shikimate pathway ( Supplementary Fig. 2 ). In order to determine the source of shikimate, we investigated whether it was present in the mice chow. We found that the chow indeed contains shikimate, and that the levels in the chow fed to SPF and GF mice are comparable (46 and 48 μM in SPF and GF mice, respectively). Further, IDA MS confirmed that the other metabolites of the shikimate pathway were not present in the chow. This suggests that the intestinal bacteria could be utilizing shikimate and depleting it from the caecum. On the other hand, the presence of O5(1-Carboxyvinyl)-3-phosphoshikimate in the GF samples suggests that the host organism may also express enzymes that can catalyse the conversion of shikimate, and that these enzymes are missing in the present annotation of the mouse genome. Similarly, we detected significant amounts of 4-amino-4-deoxychorismate in the GF samples, which could have been produced from 4-aminobenzoate via a host enzyme that is missing from the genome annotation. In contrast, chorismate, prephenate and arogenate are depleted in the GF samples, consistent with the in silico prediction, suggesting that any errors in the annotation involve enzymes that are more distal from Phe than chorismate. The physiological significance of shikimate in intestinal homeostasis warrants further investigation, since we observe shikimate to also be an activator for AhR. A logical extension of this work is to predict and identify molecules generated by the intestinal microbiota from other source metabolites under different physiologic conditions. For example, the methodology described here can be applied to identify metabolic products of emerging contaminants such as bisphenol A and phthalates, which could give rise to derivatives with either increased activity or potentially different spectrum of activity [44] . Another example is to identify metabolites derived from nutrients thought to provide benefits for gut health, such as complex carbohydrates in vegetables. In addition, predictive biomarkers could be identified for disease states such as obesity, IBD and cancer that are characterized by alterations in the GI tract microbiota [45] . A second possible extension of this work is to incorporate genomic data into the pathway analysis. In this study, we did not differentiate reactions based on their gene abundance or expression level. Consequently, each candidate reaction has an equal likelihood of selection, which is unlikely to reflect the true engagements of metabolic reactions in the gut microbiota. Metabolites produced by highly abundant organisms and/or highly expressed enzymes should more likely be present at quantifiable levels compared with the products of depleted organisms or minimally expressed enzymes. In this regard, there is an exciting opportunity to further enhance the in silico prediction step by incorporating metagenomic data, for example, from RNA-seq experiments. Our pathway construction algorithm already accepts user-specified selection weights and could be extended in a straightforward manner to explore a microbiota metabolic network weighted by relative gene abundances or expression levels. Prospectively, this type of data integration could address fundamental questions regarding not only who or what is present in the gut microbiota but also who is contributing to what function. Materials All chemicals including HPLC-grade solvents and high-purity metabolite standards were purchased from Sigma-Aldrich (St Louis, MO) unless noted otherwise. Cell culture reagents were purchased from Life Technologies (Carlsbad, CA). Microbiota metabolic network model A reaction network model of gut microbiota metabolism was constructed based on genome annotation information on select species reported to be present in the human GI tract [19] . The rationale for using human, as opposed to murine, microbiome data was that the list of documented species was more extensive. Moreover, a recent study showed that human and murine gut microbiota share a very strong similarity (90% and 89% of bacterial phyla and genera, respectively) [38] . The study by Qin et al. [19] reported a total of 194 strains with annotated genomes available in the HMP Data Analysis and Coordination Center, MetaHIT or GenBank. An organism from this list was included in the model if an exact or species-level match was found among the annotated organisms listed in KEGG because we referenced this database to map genes to enzymes to reactions. If multiple strains were listed in KEGG for a matching species, all of the strains were included, with the exception of deadly pathogens. In the case a species-level match could not be found, an organism from Qin et al. [19] was included in the microbiota model if a match was found at the genus level. In this case, the organism from Qin et al. [19] was substituted with all species listed in KEGG that belong to the same genus, provided that the species is not a deadly pathogen. Substituting for organisms with a member of the same genus ensured that the composition of the model did not significantly deviate from the current consensus on the most abundant phyla in the intestine [46] . Microbes that were matched more than once (as a result of the substitutions) were eliminated to prevent multiple entries in the final model. Out of the 194 annotated bacterial genomes referenced by Qin et al. [19] , 176 could be matched to an entry in KEGG at least at the level of genus it not species or strain. The final list of bacteria in the microbiota model comprised a total of 149 organisms, including different strains of the same species. The full list of organisms included in the microbiota model is provided in Supplementary Data 1 . A schematic outlining the steps used to assemble the microbiota reaction network model is shown in Supplementary Fig. 8 . Using a script written in MATLAB (MathWorks, Natick, MA), the KEGG enzyme database was searched for entries encoded by the genomes of the strains in the microbiota model. Each of the 6,043 enzymes in the data file was flagged as present or absent in the 149 microbiota model strains, resulting in a binary matrix E , where element e ij denotes the presence (‘1’) or absence (‘0’) of an enzyme i in species j. A similar search was then conducted through the KEGG orthology data file to generate a matrix K , where element k ij denotes the presence (‘1’) or absence (‘0’) of an orthologue group i in species j. This additional search was necessary because genome annotation in KEGG sometimes associates a gene product with a reaction without assigning an enzyme commission number (EC no.) for the reaction. On the basis of the enzyme ( E ) and orthology ( K ) matrices, corresponding reaction matrices R E and R K were generated using a text search through the KEGG reaction database. In these matrices, element r E ij or r K ij was set to 1 if enzyme or ortholog group j catalyses reaction i, and to 0 otherwise. Multiplying the enzyme or orthology matrix ( E or K ) with the corresponding reaction matrix ( R E or R K ), followed by reconciling the two matrix products (to remove duplicate entries) resulted in a matrix S specifying the metabolic reaction set available to each organism, where element s ij is a non-zero value if reaction i is catalysed by an enzyme present in organism j, and 0 otherwise. Supplementary Data 2 list the full set of microbiota model reactions and their definitions. On the basis of the reaction definitions, a corresponding set of metabolites was compiled from the KEGG compound database. The total number of reactions and metabolites in the microbiota model was 2,409 and 2,274, respectively. Uniqueness and classification of microbiota reactions The species in the microbiota model were hierarchically clustered based on the metabolic reaction sets encoded by their genomes as specified in the S matrix. For the purpose of clustering, all non-zero entries were first set to 1 to indicate the presence of the corresponding reaction in a given species. The dendrograms and heatmap ( Fig. 7 ) were generated using a built-in function (clustergram) of the Bioinformatics toolbox in MATLAB. The similarity metric and linkage type were correlation distance and average linkage, respectively. The resulting clusters of species indicated that there were metabolic functions (groups of reactions) unique to the species in a particular phylum. To determine which metabolic functions are unique to a particular subset of species or common to all species, a ‘phylum score’ was calculated as follows. 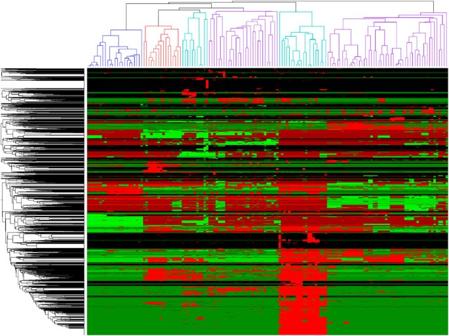Figure 7: Heat map and dendrograms show hierarchical clustering of organisms in the microbiota model based on the similarity of reaction sets encoded by their genomes. Clustering was performed on the reaction-organism matrix (S, see Methods for details), with the data standardized along the rows. Rows (reactions), and then columns (organisms), were clustered using the average linkage method based on correlation distance as the similarity metric. Colours indicate standardized row values relative to the mean. Red, black and green indicate values above, at and below the mean. Figure 7: Heat map and dendrograms show hierarchical clustering of organisms in the microbiota model based on the similarity of reaction sets encoded by their genomes. Clustering was performed on the reaction-organism matrix ( S , see Methods for details), with the data standardized along the rows. Rows (reactions), and then columns (organisms), were clustered using the average linkage method based on correlation distance as the similarity metric. Colours indicate standardized row values relative to the mean. Red, black and green indicate values above, at and below the mean. Full size image In the above equation, n j is the total number of species in phylum j, and n ij is the number of species expressing reaction i in the phylum. A score of 1 indicates that every species in a given phylum catalyses the reaction, whereas a score of 0 indicates that no species in the phylum catalyses the reaction. On the basis of these scores, each reaction in the microbiota model was classified as ‘unique’ or ‘common.’ A reaction was designated as common if the corresponding scores were >0 for more than one phylum group, otherwise designated as unique. Finally, to associate the uniqueness of reactions with metabolic function, the reactions were sorted into functional groups based on their KEGG pathway module assignments. In the case where a reaction was associated with more than one KEGG pathway modules, we used the primary assignment. Pathway analysis We used computational pathway analysis to identify possible biotransformation products of AAAs that depend on microbiota metabolism. A previously published genome-scale metabolic model of the mouse [47] was used to represent host metabolism, consistent with the experimental model used in this study. The published mouse model was manually proofread to account for any discrepancies with the most recent version of the KEGG Reaction database. After proofreading and eliminating generic reactions, the final number of unique reactions and metabolites in the mouse model were 2,182 and 2,119, respectively. This mouse model was combined with the microbiota model described above. After eliminating duplicate entries, the combined model consisted of 3,449 reactions and 3,076 metabolites, with 1,142 reactions and 1,317 metabolites present in both the mouse and microbiota. The pathway analysis used in this study built on a pathway construction algorithm previously developed to explore novel synthesis pathways for both native and non-native metabolites in a microbial metabolic engineering host [48] . For this study, we modified this algorithm to define the search space in terms of reactions, rather than metabolites. The algorithm recursively constructs a tree, starting from a user-specified source metabolite as the root of the tree. A single reaction is randomly selected from a list of candidate reactions that involve the source metabolite as a main reactant. Candidate reactions for pathway construction were drawn from the combined microbiota and host model, which represents the universe of reactions that could be expressed in the murine gut, if the models are assumed to be complete. The selected reaction is then added to the tree and represented by an edge. This edge expands the tree by attaching new nodes representing the product metabolites and cofactors of the selected reaction. The construction thus proceeds in a depth-first manner. Each of these nodes is a new root for the recursion, unless (a) the metabolite or cofactor was previously added to the tree, or (b) all reactions consuming or producing the metabolite or cofactor are present in the host (that is, mouse model). To achieve reasonable runtimes (on the order of a few minutes for a run of several thousand iterations), the size of the search space is further constrained by placing an upper limit on the number of reactions that can be used to construct a pathway. In this study, the upper limit was varied from 20 to 50, which had no observable impact on the number of the unique pathways and metabolites predicted by the algorithm. When the addition of a reaction to the tree violates the upper limit, the algorithm backtracks and proceeds by adding to the tree another reaction that has not been previously explored, effectively identifying an alternative pathway. If none of these alternative routes satisfy the pathway length limit, the algorithm further backtracks and continues from there. The algorithm finishes when all permitted-length branches of the tree terminate in a metabolite that is native to the host organism. Owing to the probabilistic nature of selecting the reactions, the completed tree does not exhaustively enumerate all possible pathways. Rather, each tree represents a single pathway from the source metabolite to one or more product metabolites that are native to the host organism. Therefore, the search is iterated many times until no more unique trees can be constructed. In our previous work, we found that the probabilistic search matches an exhaustive search in terms of sampling diversity, and dramatically outperforms the exhaustive search in terms of computational efficiency [48] . Sample collection Female C57BL/6 SPF and C57BL/6 GF mice at 6 weeks of age were purchased from Taconic (Albany, NY). The sample size ( n =7) was selected to achieve a power of at least 0.80. The power analysis was performed a priori and assumed that the s.d. was 40% of the group mean. The GF mice were shipped in a GF transport container. All mice were weighed and killed immediately upon arrival at the animal facility at Texas A&M Health Science Center. Caecum contents were collected, weighed, flash-frozen and stored at −80 °C before metabolite extraction. All animals were handled in accordance with the Texas A&M University Health Sciences Center Institutional Animal Care and Use Committee guidelines under an approved animal use protocol. Metabolite extraction Metabolites were extracted from caecum luminal contents using a solvent-based method [49] with minor modifications. Briefly, 1.5 ml of ice-cold methanol/chloroform (2:1, v/v) was added to a sample tube containing a pre-weighed luminal content or faecal sample. After homogenization on ice, the sample tube was centrifuged under refrigeration (4 °C) at 15,000 g for 10 min. The supernatant was then transferred to a new sample tube through a (70-μm) cell strainer. After adding 0.6 ml of ice-cold water, the sample tube was vortexed vigorously and centrifuged under refrigeration (4 °C) at 15,000 g for 5 min to obtain phase separation. The upper and lower phases were separately collected into fresh sample tubes with a syringe, taking care not to disturb the interface. To improve signal intensity for MS, 400 μl of the polar phase was concentrated by solvent evaporation in an Eppendorf speedvac concentrator (Eppendorf, Hauppauge, NY), and then reconstituted in 40 μl of methanol/water (1:1, v/v) for subsequent analysis. Extracted metabolites were stored at −80 °C until analysis. Multiple reaction monitoring In the case where pure chemical standards were available for purchase, metabolites were analysed using MRM to obtain absolute quantitation. We found that this MS method could provide greater sensitivity for selected metabolites compared with information-dependent acquisition (IDA) as assessed by the dynamic range of the standard curves ( Supplementary Fig. 4 ). Before sample analysis, MS parameters were optimized for each target metabolite to identify the MRM transition (precursor/product fragment ion pair) with the highest intensity under direct injection at 10 μl min −1 . The target metabolites in samples were detected and quantified on a triple quadrupole linear ion trap mass spectrometer (3200 QTRAP, AB SCIEX, Foster City, CA) coupled to a binary pump HPLC (Prominence LC-20, Shimazu, Concord, Ontario, Canada). Samples were maintained at 4 °C on an autosampler before injection. Chromatographic separation was achieved on a hydrophilic interaction column (Luna 5 μm NH 2 100 Å 250 × 2 mm, Phenomenex, Torrance, CA) using a solvent gradient method [50] . Solvent A was an ammonium acetate (20 mM) solution in water with 5% acetonitrile (v/v). The pH of solvent A was adjusted to 9.5 immediately before analysis using ammonium hydroxide. Solvent B was pure acetonitrile. Injection volume was 10 μl. The gradient method is shown in Supplementary Table 2 . Peak identification and integration were performed using the Analyst software (version 5, Agilent, Foster City, CA) to calculate the area under curve (AUC) for each metabolite identified in the polar phase. The total moles of each metabolite was calculated from standard curves and normalized to the mass of luminal contents. This quantity was divided by the density of the caecal contents (assumed to be the same as water) to determine the concentration (μM) of each metabolite in caecal luminal contents based on the fraction partitioned into the polar phase. The measured concentration is a conservative lower estimate as it does not account for either the partition of the metabolite into the non-polar phase or matrix effects resulting in ion suppression. As such, these concentration values should be interpreted as an order of magnitude estimate and was used primarily for semiquantitative comparisons between the two experimental groups. Information-dependent acquisition Pure standards could not be obtained for a large number of the metabolic derivatives identified in the pathway analysis. These metabolites were analysed using IDA experiments performed on a triple quadrupole TOF mass spectrometer (TripleTOF 5600+, AB SCIEX) coupled to a binary pump HPLC system (1260 Infinity, Agilent Technologies, Santa Clara, CA). Chromatographic separation was performed as described for the MRM experiments. Samples eluting from the column were injected into the mass analyser via a DuoSpray ion source (TurboIonSpray probe, AB SCIEX). Each sample was run twice, with the mass analyser operated in either positive or negative ion mode. The IDA method for both polarities (cycle time 650 ms) included a TOF MS (survey) scan (accumulation time: 250 ms; collision energy (CE): ±10 V) and four dependent (triggered), high-resolution MS/MS (product ion) scans (accumulation time: 100 ms each: CE, ±45 V). The TOF MS and product ion scans all had mass ranges of m/z 50 to 1,000 for both polarities. The IDA method included an automatic calibration step performed after every five samples using a polypropylene glycol solution. The identity of a detected metabolite was determined based on exact mass and isotope pattern, and, whenever possible, confirmed by comparing the calculated and measured MS/MS fragmentation patterns using PeakView (version 1.2, AB SCIEX). A difference of 30 p.p.m. was used as the tolerance threshold between the measured exact mass and the corresponding theoretical value calculated from the molecular formula. For each metabolite with a confirmed chemical identity, the corresponding peak in the chromatogram was integrated using MultiQuant (version 2.1, AB SCIEX) to determine the AUC. Fold changes in metabolite levels between different samples were calculated based on the AUC values normalized to the corresponding sample (wet caecum content) weights. Cell culture MCF-7 human breast cancer cells were obtained from ATCC (Manassas, VA). Cells were cultured at 37 °C with 5% CO 2 in RPMI 1640 medium (MP Biomedicals, Solon, OH) supplemented with 10% (v/v) fetal bovine serum, glucose (2.5 g l −1 ), HEPES (10 mM), sodium pyruvate (1 mM), sodium bicarbonate (2 g l −1 ), penicillin (100 U ml −1 ) and streptomycin (100 μg ml −1 ). Construction of GLuc reporter plasmid for AhR activation A lentiviral reporter plasmid for monitoring activation of AhR was constructed as described below. AhR response elements in target promoter were identified using the TRANSFAC database 7.0 Public. An oligonucleotide containing three repeats of the binding sequence (CTGAGGCTAGCGTGCGT) separated by four to six bases (spacer sequence) was chemically synthesized with two restriction enzyme ( EcoR I and Afe I) cleavage sites at the ends. The RE oligonucleotide was cloned into a lentiviral vector [51] in which expression of the GLuc gene is under the control of a minimal cytomegalovirus promoter and red fluorescent protein (RFP) is constitutively expressed. Expression of GLuc is induced when ligand-activated AhR binds to its RE. Clones containing the correct RE were identified by multiple restriction enzyme digests and verified by sequencing. Generation of a stable MCF-7 AhR reporter cell line A stable MCF-7 AhR reporter cell line (MCF-7/AhR-GLuc) was generated by lentiviral transduction. To produce lentiviral particles, AhR reporter plasmid and packaging plasmids psPAX (plasmid 12260, Addgene, MA) and pMD2.G (plasmid 12259, Addgene) were co-transfected into 293T/17 cells using the calcium phosphate transfection method [52] . After 24 h following the transfection, the medium was replenished and 5 mM of sodium butyrate was added. After an additional 24 h of incubation, culture supernatants containing viral particles were collected, pooled, filtered with 0.45 μm filters and centrifuged for 2 h at 4 °C at 48,000 × g . The viral titre was measured using a Lenti-X qRT-PCR titration kit (Clontech, Palo Alto, CA). To transduce MCF-7 cells, a concentrated aliquot of virus particles (~1 × 10 8 IFU) was added to the cells in presence of Polybrene (hexadimethrine bromide). After 4 h of incubation with the virus particles, the medium was replenished. AhR activation studies MCF-7/AhR-GLuc reporter cells were seeded in 24-well tissue culture plates and grown to 70% confluence. Cells were treated with indicated concentrations of target metabolites (5-hydroxy- L -tryptophan, indole, indolepyruvate, salicylate, shikimate, tryptamine, chorismate, tyramine, 3, 4-dihydroxy- L -phenylalanine and indole-3-acetate). The negative control was 0.1% (v/v) N, N -dimethylformamide and the positive controls were 20 nM TCDD and 100 μM kynurenine. For assays using the MCF-7 reporter cells, 20 μl of culture supernatant was collected at 48 h post treatment. The MCF-7 supernatant samples were stored at −20 °C until the secreted luciferase activity was measured. The luciferase activity (RLUs) was used to calculate the rate of GLuc production (RLU divided by the time over which GLuc was secreted). To account for differences in cell density between different experiments, the GLuc production rate was normalized by the intensity (relative fluorescence units) of the constitutively expressed RFP measured at 550/600 nm excitation/emission. Statistical analysis Comparisons of the medians between the metabolite levels of SPF and GF mice were performed with the non-parametric two-sided Mann–Whitney U -test. The null hypothesis that the two medians are the same was rejected for P <0.05. Comparisons of the means for the reporter experiments were performed using the Student’s t -test. The null hypothesis that the two means are the same was rejected for P <0.05. How to cite this article: Sridharan, G. V. et al. Prediction and quantification of bioactive microbiota metabolites in the mouse gut. Nat. Commun. 5:5492 doi: 10.1038/ncomms6492 (2014).